Cobweb-weaving spiders produce different attachment discs for locomotion and prey capture Spiders' cobwebs ensnare both walking and flying prey. While the scaffolding silk can entangle flying insects, gumfoot silk threads pull walking prey off the ground and into the web. Therefore, scaffolding silk needs to withstand the impact of the prey, whereas gumfoot silk needs to easily detach from the substrate when contacted by prey. Here we show that spiders accomplish these divergent demands by creating attachment discs of two distinct architectures using the same pyriform silk. A 'staple-pin' architecture firmly attaches the scaffolding silk to the substrate and a previously unknown 'dendritic' architecture weakly attaches the gumfoot silk to the substrate. Gumfoot discs adhere weakly, triggering a spring-loaded trap, while the strong adhesion of scaffolding discs compels the scaffolding threads to break instead of detaching. We describe the differences in adhesion for these two architectures using tape-peeling models and design synthetic attachments that reveal important design principles for controlled adhesion. Spiders attach their major ampullate (MA) silk dragline fibres to surfaces using attachment discs spun from pyriform silk [1] . These attachments allow spiders to move safely from place to place while secured to a dragline and to attach their webs to a variety of surfaces. Cobweb-weaving spiders spin three-dimensional webs that target both walking and flying prey [2] . While the scaffolding silk acts as a 'catching net' for flying prey, the gumfoot silk threads pull walking prey off the ground and into the web [2] , [3] . This requires that, upon agitation by the momentum of the incoming prey, the scaffolding silk remains firmly attached to the substrate while the gumfoot silk threads easily detach from the surface. Here, we show that cobweb-weaving spiders accomplish these divergent functions by creating attachment discs of two distinct architectures using the same pyriform silk. A previously known 'staple-pin' architecture is used to firmly attach the scaffolding silk to the ceiling and a newly described 'dendritic' architecture is used to weakly attach the gumfoot silk to the substrate. Interestingly, orb-weavers (evolutionary ascendants of cobweb weavers) also use the 'staple-pin' architecture to firmly attach their webs to different substrates. Peeling tests conducted on discs confirm that gumfoot dendritic discs adhere much more weakly than the scaffolding discs. We explain the difference in adhesion strengths of the two architectures by simulating the two attachment discs and using Kendall's classical tape-peeling model [4] . Small peeling angles combined with significant elastic deformation of the pyriform fibres in the scaffolding disc explain its much higher adhesion. Gumfoot discs, on the other hand, peel at much higher angles, explaining their relatively lower adhesion. These results provide unique ideas and principles for controlling structure in the design of novel tunable adhesives for various biomedical and material science applications. Different disc architectures The cobweb-weaving spider Achaearanea tepidariorum spins the same type of attachment disc used to secure scaffolding silk when it is made to walk on a glass slide and secure its dragline. Multiple pyriform gland spigots surround the MA gland spigot [5] such that the dragline silk produced by spiders is attached to surfaces using multiple nanofibres, composed of a core and a shell [6] . To sample the gumfoot disc, the spider's cage is layered with glass slides and samples are collected after the cobwebs are spun. 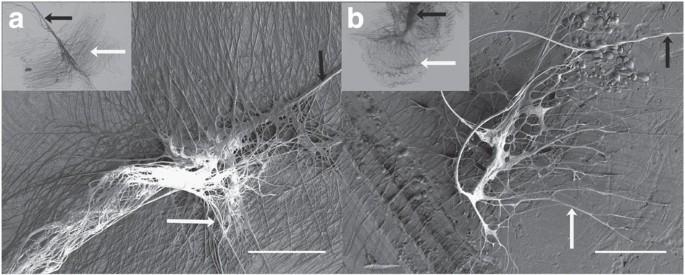Figure 1: Attachment disc morphology matches different functions. Figure shows SEM images of scaffolding discs (a) and gumfoot discs (b) spun by the cobweb-weaving spiderA. tepidariorum. Insets show optical microscope images of the respective discs. The black arrows point towards dragline silk (MA silk) in (a) and its inset, while the white arrows point towards pyriform fibres, arranged in a 'staple-pin' architecture, attaching the dragline silk to the surface. Black arrows point towards gumfoot thread (MA silk covered with aggregate glue) in (b) and its inset, while the white arrows point towards pyriform fibres, arranged in a dendritic architecture, attaching the gumfoot thread to the surface. Scale bars in both the figures are 100 μm. Figure 1 shows SEM micrographs of the scaffolding disc and the gumfoot disc. The difference in the architectures of the discs is clear. The scaffolding disc resembles a 'staple-pin' architecture, while the gumfoot disc shows a 'dendritic' architecture. Each pyriform fibre is coated with a fluid that likely facilitates adhesion to both smooth and rough surfaces ( Supplementary Fig. S1 ). The number of pyriform fibres in staple-pin discs is much higher than in dendritic discs (1,550±100 versus 188±20), which translates into a greater number of load-bearing attachment points in staple-pin discs. (There are observable intra-species differences in the size of the joints and the density of pyriform fibres within each joint. To avoid these differences, the numbers were calculated using gumfoot and scaffolding joints spun by the same spider). Moreover, in gumfoot discs, pyriform fibres are suspended in the air as they converge with gumfoot threads and are bound to the surface only at the periphery of the discs ( Supplementary Fig. S2 ). This results in only the thinnest pyriform fibres contacting the surface, as pyriform fibres bifurcate successively, becoming thinner towards the periphery of the discs ( Supplementary Fig. S2 ). In contrast, in scaffolding discs, most of the length of the pyriform fibres, which are thicker than in gumfoot discs, is in contact with the surface. Figure 1: Attachment disc morphology matches different functions. Figure shows SEM images of scaffolding discs ( a ) and gumfoot discs ( b ) spun by the cobweb-weaving spider A. tepidariorum . Insets show optical microscope images of the respective discs. The black arrows point towards dragline silk (MA silk) in ( a ) and its inset, while the white arrows point towards pyriform fibres, arranged in a 'staple-pin' architecture, attaching the dragline silk to the surface. Black arrows point towards gumfoot thread (MA silk covered with aggregate glue) in ( b ) and its inset, while the white arrows point towards pyriform fibres, arranged in a dendritic architecture, attaching the gumfoot thread to the surface. Scale bars in both the figures are 100 μm. Full size image Attachment discs are formed without the involvement of legs [7] , so differences result solely from movements of the abdomen and spinnerets. The anterior spinnerets are brought into direct contact with the substrate and are rubbed against it while a secretion is exuded through the pyriform gland spigots [7] . The different architectures of the attachment discs therefore imply different movement patterns of the anterior spinnerets against the substrate. Based on high-resolution images of the discs, and the hairpin bends as shown in Supplementary Fig. S1 , we postulate that the spinnerets 'sweep' back and forth across an MA fibre several times to create a scaffolding disc, whereas the successive splitting of the pyriform fibres in the gumfoot disc ( Supplementary Fig. S2 ) indicates that the anterior spinneret rubs against the substrate once, going inwards from the periphery of the gumfoot disc. This also implies that the pyriform fibres are not completely solidified when secreted and that they coalesce to form thicker fibres, going inwards from the periphery of a gumfoot disc. Incidentally, cribellate spiders also use nanofibres for adhesion [8] . However, unlike in pyriform fibres, these nanofibres are drawn from the cribellum of the spiders by a setal comb on their legs [8] . Moreover, the cribellar fibres solidify upon drawing, as indicated by their uniform diameter, unlike pyriform fibres. Effect of architecture on adhesion To determine the effect of architecture on attachment strength, the discs were peeled from a clean glass surface at a controlled rate, by pulling on the dragline silk/gumfoot silk thread perpendicular to the plane of the respective discs. Interestingly, scaffolding discs (for both cob- and orb-webs) could not be induced to peel from glass by pulling the underlying dragline silk vertically. Instead, the dragline silk thread itself always failed before peeling of the scaffolding discs was completed. This demonstrates that the adhesion force of the scaffolding discs is greater than the breaking force of MA silk (dragline silk), which is the strongest (highest breaking force) silk used in the web. Spiders were hence made to spin scaffolding discs on glass slides laid across a much thicker nylon thread (30 μm diameter) ( Fig. 2a ), to test the discs' maximum adhesive strength. Using the nylon thread, a scaffolding disc was peeled as shown in the Supplementary Movie 1 . The pyriform threads deform and peel sequentially, starting from one end of the disc, at low peeling angles leading to eventual fracture. 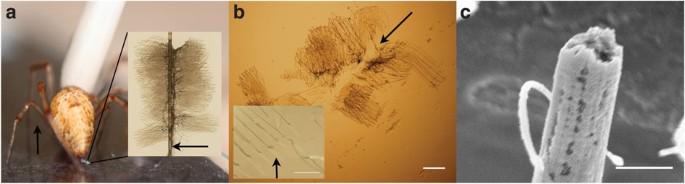Figure 2: Scaffolding disc adhesion testing. (a) Shows the cobweb-weaving spiderA. tepidariorumspinning a scaffolding disc on a nylon thread. The inset shows an optical microscope image of a scaffolding disc spun on a nylon thread (30 μm diameter). The black arrows point towards the nylon thread in both (a) and its inset. (b) Shows a scaffolding disc post peeling. The black arrows in (b) and its inset point towards the peeling zone of the scaffolding disc spun on a nylon thread. Pyriform fibres peel a certain distance followed by breaking, as is shown in the inset. The scale bar in (b) and its inset is 100 μm and 25 μm, respectively. (c) Shows a broken pyriform fibre from a scaffolding disc that has been peeled. The scale bar is 1 μm. Figure 2b shows the post-peeling SEM picture of a scaffolding disc spun on a nylon thread. An SEM micrograph of broken pyriform fibre from the scaffolding disc is shown in Fig. 2c . Figure 2: Scaffolding disc adhesion testing. ( a ) Shows the cobweb-weaving spider A. tepidariorum spinning a scaffolding disc on a nylon thread. The inset shows an optical microscope image of a scaffolding disc spun on a nylon thread (30 μm diameter). The black arrows point towards the nylon thread in both ( a ) and its inset. ( b ) Shows a scaffolding disc post peeling. The black arrows in ( b ) and its inset point towards the peeling zone of the scaffolding disc spun on a nylon thread. Pyriform fibres peel a certain distance followed by breaking, as is shown in the inset. The scale bar in ( b ) and its inset is 100 μm and 25 μm, respectively. ( c ) Shows a broken pyriform fibre from a scaffolding disc that has been peeled. The scale bar is 1 μm. Full size image To quantify the adhesion of gumfoot discs, the discs were peeled by pulling on the lower region of the gumfoot thread, which is composed of four MA fibres [2] . To sample the gumfoot discs for adhesion measurements, the spider cages were layered with glass slides such that after the webs were spun, a flag, like that shown in Fig. 3a , was used to collect the gumfoot silk thread with the attachment disc undisturbed. 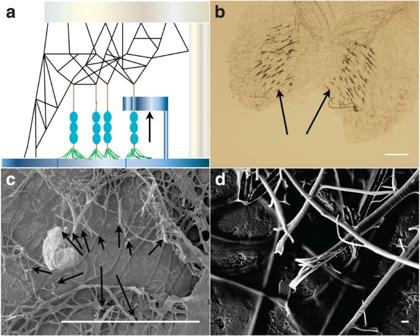Figure 3: Gumfoot disc adhesion testing. (a) Shows a schematic of a typical cobweb. The black arrow points towards the flag used to collect individual gumfoot threads with the attached pyriform attachment disc (light green). (b) Shows a gumfoot disc post peeling. The picture shows a fibre-dense two-lobed structure, Scale bar is 50 μm. (c) and (d) show SEM images of a gumfoot disc post fracture. Black arrows indicate broken pyriform fibres. The scale bars are 100 μm and 1 μm, respectively. Figure 3b,c show an optical image and an SEM micrograph of a gumfoot disc, post peeling. The fracture image shows two fibre-dense 'lobes' in the gumfoot discs. Figure 3d shows an SEM micrograph of broken pyriform fibres from the gumfoot disc. The diameters of the broken end of the pyriform fibres in both scaffolding and gumfoot discs are similar. Supplementary Movie 2 shows the behaviour of pyriform fibres during peeling of a gumfoot disc. Depending on the angle at which the gumfoot thread is pulled, pyriform fibres in the two 'lobes' behave differently. The peeling angles of gumfoot fibres are much higher than the peeling angles in scaffolding discs. Also, unlike in scaffolding discs where pyriform fibres deform and peel sequentially from one side of the disc, in gumfoot discs, all the pyriform fibres respond simultaneously. Figure 3: Gumfoot disc adhesion testing. ( a ) Shows a schematic of a typical cobweb. The black arrow points towards the flag used to collect individual gumfoot threads with the attached pyriform attachment disc (light green). ( b ) Shows a gumfoot disc post peeling. The picture shows a fibre-dense two-lobed structure, Scale bar is 50 μm. ( c ) and ( d ) show SEM images of a gumfoot disc post fracture. Black arrows indicate broken pyriform fibres. The scale bars are 100 μm and 1 μm, respectively. 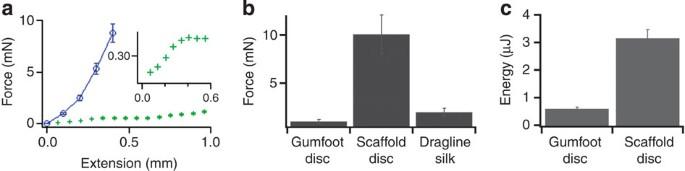Figure 4: Adhesion measurements. (a) Shows the force-extension curves obtained by peeling the scaffolding discs (blue) and gumfoot discs (green) spun on a clean glass surface. Data are plotted as mean±s.d. from three measurements each. Inset emphasizes the initial region of the force-extension curve of the gumfoot disc. (b) Shows the force required to separate a gumfoot disc and a scaffolding disc from a clean glass surface. Gumfoot disc adhesion is an order weaker than scaffolding disc adhesion. The force required to break a dragline silk (MA silk) thread is also plotted. A dragline silk thread breaks when it is pulled to peel a scaffolding disc (hence thicker nylon threads were used to peel scaffolding discs). Gumfoot discs were peeled using the gumfoot silk threads (four intertwined MA threads). Data are plotted as mean±s.d. from five measurements each. In theory, however, gumfoot discs could be peeled using just one MA thread as the breaking force of MA thread is almost twice the pull-off force of gumfoot discs with glass. This indicates that scaffolding disc adhesion is much stronger than gumfoot disc adhesion. (c) Shows the energy of adhesion of a gumfoot disc and a scaffolding disc. Gumfoot discs adhere an order weaker than scaffolding discs adhere. The energy of adhesion is determined by subtracting the strain energy contribution of nylon threads (while peeling scaffolding discs) and gumfoot threads (while peeling gumfoot discs) from the total work done in peeling the discs. Data are plotted as mean±s.d, from five measurements each. Full size image Figure 4a shows the force-extension behaviour obtained from peeling scaffolding and gumfoot discs spun on clean glass surfaces. The maximum force required to peel the discs is considered the 'adhesion force' or the 'pull-off force'. Figure 4b compares the pull-off forces of the discs on glass. Scaffolding discs bind by an order of magnitude stronger than in gumfoot discs. The total work done in peeling the discs can be calculated by integrating the area from the force-displacement results. The total work done involves work incorporated in stretching the thread (nylon in the case of scaffolding discs) and the energy expended in peeling the discs. The strain energy stored in nylon threads and gumfoot silk threads was independently determined from tensile stress-strain measurements and was subtracted from the total work done (calculated by integrating the area under the force-extension curve obtained from the disc peeling measurements) to calculate the work done owing to peeling (as shown in Fig. 4c ) for scaffolding discs and gumfoot discs, respectively. Scaffolding discs adhere much more strongly than gumfoot discs, as anticipated. The work done owing to peeling comprises of stretching, separating and breaking of pyriform fibres, as shown by high-speed videos taken during peeling, and should thus, in theory, be much higher than the thermodynamic work of adhesion of pyriform fibres. Figure 4: Adhesion measurements. ( a ) Shows the force-extension curves obtained by peeling the scaffolding discs (blue) and gumfoot discs (green) spun on a clean glass surface. Data are plotted as mean±s.d. from three measurements each. Inset emphasizes the initial region of the force-extension curve of the gumfoot disc. ( b ) Shows the force required to separate a gumfoot disc and a scaffolding disc from a clean glass surface. Gumfoot disc adhesion is an order weaker than scaffolding disc adhesion. The force required to break a dragline silk (MA silk) thread is also plotted. A dragline silk thread breaks when it is pulled to peel a scaffolding disc (hence thicker nylon threads were used to peel scaffolding discs). Gumfoot discs were peeled using the gumfoot silk threads (four intertwined MA threads). Data are plotted as mean±s.d. from five measurements each. In theory, however, gumfoot discs could be peeled using just one MA thread as the breaking force of MA thread is almost twice the pull-off force of gumfoot discs with glass. This indicates that scaffolding disc adhesion is much stronger than gumfoot disc adhesion. ( c ) Shows the energy of adhesion of a gumfoot disc and a scaffolding disc. Gumfoot discs adhere an order weaker than scaffolding discs adhere. The energy of adhesion is determined by subtracting the strain energy contribution of nylon threads (while peeling scaffolding discs) and gumfoot threads (while peeling gumfoot discs) from the total work done in peeling the discs. Data are plotted as mean±s.d, from five measurements each. Full size image The differences in pull-off forces can be attributed to differences in the number, diameter, chemistry (intrinsic adhesion strength) and the peeling angles of the pyriform fibres between these two discs. To test the effect of number of fibres, we controlled the length of the scaffolding disc as shown in Fig. 5a–g and measured the pull-off forces as a function of number of fibres ( Fig. 5h ). The pull-off force initially increases with the number of pyriform fibres and then plateaus for higher numbers of fibres. The plateau in pull-off forces is expected because in the staple-pin architecture only a few fibres resist the pull-off forces at a time since the peeling starts from one end of the disc and the deformation zone is smaller than the scaffolding disc. Interestingly, for the same number of fibres in the scaffolding and gumfoot discs, the pull-off force of the scaffolding disc is almost six times that of the gumfoot disc ( Fig. 5h ). Moreover, scaffolding discs with fewer than half the number of fibres in a gumfoot disc still generate a pull-off force three times as big. Therefore, the differences in the pull-off forces between the scaffolding and gumfoot discs cannot be solely caused by the differences in the number of pyriform threads. The SEM images of the broken fibres in both the discs ( Figs 2c and 3d ) suggest that the effect also cannot be explained by differences in diameters of the fibres. Instead, scaffolding discs generate high pull-off forces owing to their architectures. 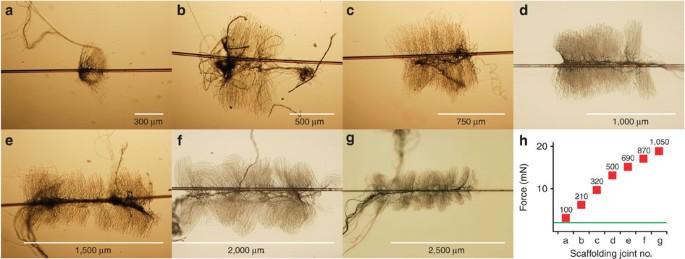Figure 5: Effect of number of fibres on scaffolding disc adhesion. (a–g) Show scaffolding discs spun on nylon thread containing 100, 210, 320, 500, 690, 870 and 1,050 pyriform fibres, respectively. (h) Shows the adhesion forces of these discs. The green line shows the breaking force of an MA thread, which, as shown inFig. 4b, is higher than the adhesion force of a gumfoot disc. Figure 5: Effect of number of fibres on scaffolding disc adhesion. ( a–g ) Show scaffolding discs spun on nylon thread containing 100, 210, 320, 500, 690, 870 and 1,050 pyriform fibres, respectively. ( h ) Shows the adhesion forces of these discs. The green line shows the breaking force of an MA thread, which, as shown in Fig. 4b , is higher than the adhesion force of a gumfoot disc. Full size image To test the possibility that the pyriform fibres in the scaffolding and gumfoot discs could be chemically different, we cite the work of Moon et al . [9] that shows that female A. tepidariorum spiders possess 90–100 pairs (total 180–200) of pyriform glands that feed into discrete pyriform spigots on the anterior spinnerets. The total number of pyriform spigots is consistent with the total number of fibres measured by us in the gumfoot discs (188±20). Also, the number of pyriform fibres in scaffolding discs is 1,550±100 (which, we hypothesize, result from several strokes of spider's abdomen across an MA thread). This suggests that all the pyriform glands are employed for creating gumfoot discs, and hence the scaffolding and gumfoot discs are spun by the same spinnerets and thus have the same chemistry. This also implies that the difference in the pull-off forces of the gumfoot and scaffolding discs is not due to difference in chemistry. The remaining hypothesis we put forth to explain the differences in the pull-off forces is the differences in the peeling angles (as shown in Supplementary Movies 1 and 2 ). The effects of peeling adhesive tapes as a function of peeling angles was studied by Kendall [4] , [10] and he showed that peeling force at low peeling angles depend on the modulus of the fibres and physical factors such as width and thickness of the tape. At higher peeling angles, the pull-off forces were considerably lower and they only depended on the adhesion energy (referred to here as fracture energy, G ) and the width of the tape. Therefore, we anticipate that the peeling angles could explain the differences in pull-off forces between the two different architectures of attachment discs used by spiders. Synthetic joints inspired by pyriform attachment discs We design two models using adhesive tapes to illustrate the differences in the architecture used in these two attachment discs. These macroscopic models also allow us to understand the functional implications of materials used by spiders and test conditions that we could not control in these natural materials. A scaffold disc is modelled by attaching a bundle of nylon fibres on a clean glass surface using six strips of a stretchable tape (3 M , MMM8884) perpendicular to the long axis of the strand ( Fig. 6a ). Peeling of the tape strips is induced by pulling on the 'peeling end' of the nylon strand perpendicular to the plane of the tapes, at a fixed rate (inset, Fig. 6a ). The rate of pulling is kept fixed throughout the study because the fracture energy G , and hence the peeling force F , depend on the rate. 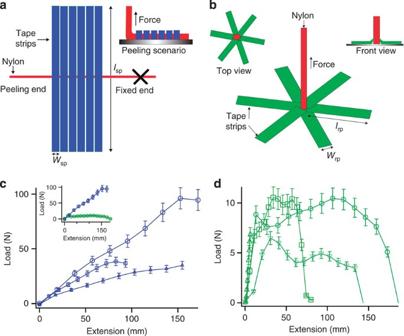Figure 6: Modelling attachment discs. (a) Shows a schematic of the simulated scaffolding disc. The lengthlspis 100 mm while the widthwspis such that 6*wspequals 36 mm. The inset shows how the peeling measurements are conducted. The nylon strand is pulled on perpendicular to the plane of the tapes while the load-extension behaviour is registered. (b) Shows a schematic of the simulated gumfoot disc. The lengthlrpand the widthwrpof the tape strips are equal tolspandwsp, respectively. All six strips are firmly secured to the strand of nylon threads at the centre of the circle. The insets on the left and right show the top and front views, respectively, of the modelled tapes. (c) Shows the load-extension results obtained from the adhesion measurements of the simulated scaffolding discs. Circles denote the case with length=lspand widthwsp, squares with length=lsp/2 and width=wsp, and triangles with length=6*wspand width=lsp. The inset shows a plot comparing the adhesion forces of simulated scaffolding silk with the simulated gumfoot disc, both using the same dimensions of the strip: length=lsp, width=wsp. (d) Shows the load-extension results obtained from the adhesion measurements of the simulated gumfoot discs. Circles denote the case with lengthlrpand widthwrp. Squares denote length ~lrp/2 and widthwrp, inverted triangles denote lengthlrp*3/4 and widthwrp/2, and upright triangles denote widthwrpand length ~3 mm. For (c) and (d), data are plotted as mean±s.d. from five measurements each. Figure 6: Modelling attachment discs. ( a ) Shows a schematic of the simulated scaffolding disc. The length l sp is 100 mm while the width w sp is such that 6* w sp equals 36 mm. The inset shows how the peeling measurements are conducted. The nylon strand is pulled on perpendicular to the plane of the tapes while the load-extension behaviour is registered. ( b ) Shows a schematic of the simulated gumfoot disc. The length l rp and the width w rp of the tape strips are equal to l sp and w sp , respectively. All six strips are firmly secured to the strand of nylon threads at the centre of the circle. The insets on the left and right show the top and front views, respectively, of the modelled tapes. ( c ) Shows the load-extension results obtained from the adhesion measurements of the simulated scaffolding discs. Circles denote the case with length= l sp and width w sp , squares with length= l sp /2 and width= w sp , and triangles with length=6* w sp and width= l sp . The inset shows a plot comparing the adhesion forces of simulated scaffolding silk with the simulated gumfoot disc, both using the same dimensions of the strip: length= l sp , width= w sp . ( d ) Shows the load-extension results obtained from the adhesion measurements of the simulated gumfoot discs. Circles denote the case with length l rp and width w rp . Squares denote length ~ l rp /2 and width w rp , inverted triangles denote length l rp *3/4 and width w rp /2, and upright triangles denote width w rp and length ~3 mm. For ( c ) and ( d ), data are plotted as mean±s.d. from five measurements each. Full size image The gumfoot discs are simulated by placing six strips of the same tape in a radial pattern, such that all the strips are securely attached to a strand of nylon threads at the centre of the circular disc ( Fig. 6b ). Here, peeling of the tapes is induced by pulling the nylon strand perpendicular to the plane of the tapes, at a fixed rate. Figure 6c,d shows the adhesion forces of both geometries. For the same surface area of the tape, the 'staple-pin' geometry (mimicking scaffolding discs) requires a much larger force to detach than the dendritic geometry (mimicking gumfoot discs) (blue circles versus green circles and blue squares versus green squares, Fig. 6c,d ). The energy expended (area under the load-extension curve) is also higher for the 'staple-pin' geometry. Peeling the modelled scaffolding disc involves deformation of the tape strips and their concomitant detachment from the glass surface. The detachment of the tape from the glass surface follows a near-zero degree peeling behaviour, with a small gradual increase in peeling angle during further peeling. Consistent with Kendall's observations with tapes, the thickness of the tape strips, d , affects the fracture energy of the simulated scaffolding disc ( Supplementary Fig. S3a , solid blue squares). Detachment of simulated gumfoot discs, however, initiates as a near-ninety degree tape peeling, the peel angle reducing only slightly during further peeling. The testing method for both the modelled discs involved slight changes in the peeling angle during the course of peeling. This was done to simulate the real-life scenario and also the method used to test the natural attachment discs). In the radial peeling of six-tape strips of width w rp , each was observed to be equivalent to peeling of a single tape strip of width 6* w rp . Each curve shows a 'fracture-initiation region,' followed by a 'fracture-propagation region.' The propagation region scales with the width of the tape: a tape of width < w rp shows a propagation region of smaller magnitude (inverted triangles, Fig. 6d ), while a shorter tape of the same width has a propagation region of the same magnitude (squares, Fig. 6d ). Successively reducing the length of the tape, keeping width constant, results in the extreme case where just the initiation region is observed: fracture propagation is absent (green upright triangles, Fig. 6d ). Also, varying the thickness of the tape has no effect on radial peeling, unlike in the staple-pin case, consistent with Kendall's observations (green solid squares, Supplementary Fig. S3b ). The slight increase in the propagation regions of all the curves is explained by the small reduction in peeling angle during peeling. To accomplish peeling of the modelled discs, a nylon strand of breaking force ≫ 200 N was used. In reality, however, MA silk thread breaks before peeling of the scaffolding discs. This was simulated by using a thinner strand of nylon threads (breaking strength ~60 N). Using this strand, the simulated gumfoot disc still peels completely, but an attempt to peel a simulated scaffolding disc instead causes fracture of the nylon strand before the disc detaches. These simulation results clearly demonstrate the design principles employed by spiders to make strong versus weak discs using the same material. Why do spiders create two different architectures for attachment discs? The difference in pull-off forces for these two divergent architectures has major implications on locomotion and prey capture by spiders. When an insect encounters an orb-web (which is also attached to different surfaces using pyriform discs spun in the staple-pin architecture), the hysteretic behaviour of the MA fibres, as they stretch and relax, accounts for majority of the energy absorbed by the web [11] . Also, when an insect becomes completely entangled, the weight of the insect is supported by the MA fibres, transferring the load to the attachment points of the web with the surface. Stiffness, strength, toughness and viscoelasticity of the MA silk are key to the functioning of both the orb and cobwebs. However, the excellent properties of MA silk can only be utilized for capturing prey if the threads are firmly fixed to surfaces. Spiders accomplish this by creating attachment discs out of pyriform silk that have 'staple-pin' architectures. The observation that the pull-off forces of these discs are higher than the breaking strength of MA silk has major implications for optimized web engineering: the mass and velocity of the incoming prey are limited solely by the breaking strength of the strong MA silk and not by its attachment to surfaces. In contrast, the gumfoot discs are attached very weakly to the substrate, which enables the gumfoot threads to detach easily. Energy stored in the scaffolding silk suspends the insect helplessly in the air. A gumfoot thread is composed of four MA silk threads at its base [2] . During adhesion measurements, gumfoot discs could be easily peeled from a surface by vertically pulling the gumfoot thread attached to the discs. The pull-off force of a gumfoot disc is ~50% the breaking force of one MA silk thread (~1/8th the breaking strength of a gumfoot thread, as there are four MA threads in the lower region of a gumfoot thread). A macroscopic tape model ( Fig. 6 ) illustrates not only the importance of peeling angles in controlling pull-off forces but also the requirement for the gumfoot discs to act as an efficient trap: discs should release with ease only after being agitated by an insect. Gumfoot threads are spring-loaded traps always held in tension. These traps are triggered when agitated by a walking insect. An ideal trap acts spontaneously upon triggering by prey, but not upon minor perturbations of the web owing to wind or even the spider moving through its own web. We postulate that the initial over-shoot region acts as a trigger, going past the region in which the propagation region slopes downwards ( Supplementary Fig. S3b , green diamonds). Once the agitation force caused by the insect surpasses the initial over shoot, the gumfoot discs rapidly release with ease, suspending the insect helplessly in the air for the spider to subdue. The force profile during peeling of a staple-pin disc instead slopes upwards continuously, which is ideal for developing a strong disc that resists catastrophic failure but it does not fulfil the trigger requirement of an ideal spring-loaded trap. The force-extension profiles demonstrated by the tape models mimic those measured in actual scaffolding and gumfoot discs ( Fig. 4a ). The Kendall model for elastic adhesive tapes of width ' w ', the peeling force for large peeling angle ( θ ) is equal to w * G /(1−cos( θ )), where G is the fracture energy. After the initial zone, the peeling force should be independent of the length of the tape (or length of pyriform fibres in dendritic discs). In addition, the force should be proportional to the width (or the diameter of the thread). Therefore, in the tape model, varying the amount of material in a gumfoot disc does not change the maximum force required to peel the disc ( Fig. 6d , green circles and green squares). In the actual gumfoot discs, fibres in contact with the surface are mostly at the periphery of the disc and become successively thinner going towards the periphery ( Supplementary Fig. S2 ), which is most accurately modelled by using tapered strips of tape represented by green diamonds in Supplementary Fig. S3b . As the peeling force is a function of width, the progressively thinner diameter insures that there will be a quick release of the thread. Another interesting design parameter used in spinning the staple-pin architecture is the width of the attachment disc. The lengths of the pyriform fibres are 250 times the diameter of the secured MA silk thread (~1,000 μm versus 4 μm), which seems to suggest that a lot of 'expensive material' used to spin pyriform fibres is wasted, and that pyriform secretions could either have been saved or used to cover a longer length of MA silk thread with shorter pyriform fibres. We tested these conditions using the tape model to illustrate the importance of the width of the attachment disc ( Fig. 6c ). Keeping the width of each strip constant ( w sp ), if the length of each strip is reduced to l sp /2 (so that the volume of tape is essentially halved), the adhesion force is reduced by almost 50% (blue squares versus blue circles, Fig. 6c ). In contrast, using the same volume of the material to produce wider strips of width l sp /6, where length is reduced to 6* w sp (blue triangles, Fig. 6c ) reveals an interesting behaviour: even though the length of the nylon strand covered by the tape to immobilize it on the glass surface is now much longer, that is, l sp compared with the previous value of 6* w sp , the force and energy required to detach is smaller by 50%. Interestingly, this value is even lower than when 50% of the material (length of each strip= l sp /2) was used (blue triangles versus blue squares, Fig. 6c ). Thus, for a given volume of material more adhesion is generated by covering a shorter length of dragline with long and thin pyriform fibers. During staple-pin peeling, the tape strips have to be deformed for the fracture to initiate and propagate. In the first case (width w sp and length l sp ), peeling requires higher force to deform and detach the longer strips of length l sp . However, in the third case (width l sp /6 and length 6* w sp ), much smaller force is required because the length to be deformed and detached is only 6* w sp . This might explain why spiders use long fibres (higher disc width) to make the scaffolding disc. The pull-off forces in these studies were measured on a clean glass surface, which is a simplified perspective considering that the spiders attach to rough surfaces, including wood, leaves and even concrete. Based on our measurements ( Fig. 4 ) and our field observations, it appears that scaffolding disc always adheres more strongly than the force required to break the MA silk thread. However, the gumfoot disc adhesion depends on the surface, for example, they fracture cohesively on a clean glass surface (green curve, Figs 4a and 3a,b ), but fracture adhesively on a hydrophobic surface. The successive bifurcation of glue threads ( Supplementary Fig. S2 ) would either facilitate breaking or precipitate detachment through peeling depending on the surface. In summary, the cobweb-weaving spiders exploited the difference in architecture of the attachment discs, rather than the chemistry of the silk, to achieve either a very strong attachment of the discs to hold the dragline permanently to substrates or controlled attachment points that release rapidly when contacted by prey. This is further demonstrated by studying the attachment discs of the evolutionary ascendants of cobweb-weaving spiders, the orb-weaving spiders. The orb-weavers also use 'staple-pin' architecture to firmly attach their orb-webs to different surfaces, similar to how cobweb weavers attach their scaffolding sheet to a variety of surfaces ( Supplementary Fig. S4 ) ( Supplementary Fig. S4 shows a disc spun by the furrowed orb-weaver Larinioides cornutus . Their distant relatives, Nephila clavipes , also spin discs with the same structure, indicating the prevalence of this structure among orb-weavers. Similarly, black widow spiders, Latrodectus hesperus , also spin both staple-pin and dendritic discs, indicating the prevalence of the architecture philosophy among cobweb weavers.). The chemical composition of the proteins in the pyriform silk for orb-weavers differs from the cobweb weavers [12] . However, just like the scaffolding discs of cobweb-weavers, the adhesion of orb-weaver's staple pin discs is higher than the breaking force of their MA thread, emphasizing the importance of the architecture rather than the differences in the chemical composition of the pyriform silk. Our models show that this variation in pull-off forces and behaviour does not require specialization of the chemistry in the glues, but is clearly controlled by architecture. It is now recognized that the spinning process is very important in achieving high tensile strength, super contractibility and other excellent properties of silk [13] , [14] , [15] . Here, we emphasize how spiders also use the architecture of attachments to control pull-off forces and detachment behaviour. These results provide design principles of using synthetic adhesives to fabricate tunable structural adhesives by using the known chemistry available today. Disc sample preparation Scaffolding disc samples were produced by making the spider ( A. tepidariorum, L. cornutus, L. hesperus or N. clavipes) walk on a clean glass slide layered with a single nylon thread (diameter 30 μm) such that the spider spun the scaffolding disc symmetrically to the nylon fibre ( Fig. 2b ). For making discs of a desired length, a blade was used to remove the extra pyriform fibres from that disc. Gumfoot disc samples were prepared by layering a cobweb-weaver's cage with glass slides and using a flag ( Fig. 3a ) to collect the gumfoot samples with the gumfoot disc. To acquire an SEM image (JEOL) of the discs, spiders were made to walk and spin a disc on an SEM stub, and for the gumfoot disc case, the cages were layered with SEM stubs. Adhesion testing on discs Nylon threads used for the scaffolding disc were fixed on the top clamp of a NanoBionix (Agilent Tech.) while the glass slide with the scaffolding disc was fixed on the bottom clamp. The nylon thread was pulled perpendicular to the plane of the disc at 2 mm s −1 while the load-extension behaviour was recorded. To test the gumfoot disc, gumfoot threads were fixed on the top clamp, and the glass slide with the gumfoot disc was fixed on the bottom clamp. The gumfoot thread was pulled perpendicular to the plane of the disc at 2 mm s −1 while the load-extension behaviour was recorded. Adhesion testing on simulated discs Strips of a stretchable tape (3 M, MMM8884) were used to attach a strand of nylon threads to a clean glass plate in the manner described in the text and shown in Fig. 6a,b . For the adhesion testing, the glass plate was fixed on the bottom clamp of an Instron, and the nylon strand was fixed on the top clamp. The nylon strand was pulled perpendicular to the plane of the tape strips at a rate of 50 mm min −1 while the load-extension behaviour was recorded. How to cite this article: Sahni, V. et al . Cobweb-weaving spiders produce different attachment discs for locomotion and prey capture. Nat. Commun. 3:1106 doi: 10.1038/ncomms2099 (2012).